Autophagy supports genomic stability by degrading retrotransposon RNA Many cytoplasmic substrates degraded by autophagy have been identified; however, the impact of RNA degradation by autophagy remains uncertain. Retrotransposons comprise 40% of the human genome and are a major source of genetic variation among species, individuals and cells. Retrotransposons replicate via a copy-paste mechanism involving a cytoplasmic RNA intermediate. Here we report that autophagy degrades retrotransposon RNA from both long and short interspersed elements, preventing new retrotransposon insertions into the genome. Retrotransposon RNA localizes to RNA granules, whose selective degradation is facilitated by the autophagy receptors NDP52 and p62. Accordingly, NDP52 and p62 control retrotransposon insertion in the genome. Mice lacking a copy of Atg6/Beclin1 , a gene critical for autophagy, also accumulate both retrotransposon RNA and genomic insertions. Thus, autophagy physiologically buffers genetic variegation by degrading retrotransposon RNA. This may contribute to the increased tumorigenesis occuring when autophagy is inhibited and suggest a role for autophagy in tempering evolutionary change. Stress instigates cellular programs for adaptation. Critical among these is macroautophagy (hereafter referred to as autophagy), a mechanism of cytoplasmic degradation. In autophagy, a double membrane is formed de novo in the cytoplasm and expands to engulf cytoplasmic contents, eventually enclosing them within an autophagosome [1] . Lysosomes subsequently fuse with autophagosomes delivering catabolic enzymes including RNAses [1] . Autophagy can selectively degrade cytoplasmic content using autophagy receptors, such as NDP52 or p62 (official gene symbols CALCOCO2 and SQSTM1, respectively), which recruit selective cargo to the nascent autophagosome membrane [2] . While the field of autophagy has focused on proteins and organelles degraded by autophagy, only recently has attention shifted to RNA degradation by autophagy [3] , [4] . Retrotransposons, ancient symbionts whose genetic material is sheltered and replicates within the human genome [5] , [6] , [7] , [8] , are a major contributor to genetic variation between species, within species and between cells in a single individual. Two of the principal families of retrotransposons, long interspersed nucleotide elements (LINE-1) and short interspersed nucleotide elements, such as the dominant Alu family in primates, account for 17 and 10% of the human genome, respectively [9] . By reinserting themselves in the genome, retrotransposons drive genetic change but also cause over 65 diseases identified to date [9] . Increasing attention is therefore being devoted to mechanisms that control retrotransposon insertions and balance the risks of unhindered retrotransposon replication with their potentially adaptive benefits [10] . Both Alu and LINE-1 replicate using a copy-paste mechanism requiring two proteins encoded by LINE-1: ORF1p and ORF2p (ref. 5 ). RNA is transcribed from genome-integrated copies of retrotransposons and transits through the cytoplasm [11] . ORF1p is required for retrotransposition and binds LINE-1 and Alu RNA in the cytoplasm [12] . Retrotransposon RNA traffics back into the nucleus where ORF2p copies and reinserts the retrotransposon in a new genomic location [5] . Our understanding of the spectrum of mechanisms quelling retrotransposons is limited, but retrotransposon RNA is susceptible to repression during transit through the cytoplasm [13] . Here we demonstrate that autophagy degrades LINE-1 RNA and tempers the rate of insertion of LINE-1 and Alu retrotransposons by using the autophagy receptors NDP52 and p62 to target P-bodies and stress granules for elimination. Our evidence suggests that this mechanism causes genetic changes in select tissues of mice lacking a copy of Atg6/Becn1 , a gene critical for autophagy. Retrotransposon RNA co-localizes with autophagosomes If LINE-1 and Alu RNA are degraded by autophagy, they should co-localize, in part, with autophagosomes. To visualize the subcellular localization of LINE-1 RNA, as previously described [11] , we co-expressed LINE-1 RNA fused with six MS2-binding sites (LINE-1-MS2) and MS2-green fluorescent protein (GFP). As described, LINE-1-MS2 accumulated in cytoplasmic foci [11] , 65% of which co-localized with a specific ( Supplementary Fig. 1a–c ) autophagosome marker LC3 ( Fig. 1a,b ). Similarly, foci of Alu -MS2 RNA detected with the MS2-GFP system co-localized with LC3 ( Fig. 1c ). Consistent with autophagic elimination of LINE-1-MS2 RNA, the number of foci of LINE-1-MS2 increased when degradation of autophagosome content was blocked with Bafilomycin A1 (BAF; Fig. 1d ). The number of foci of LINE-1-MS2 RNA that co-localized with the autophagosome marker, LC3, also increased when autophagic degradation was inhibited ( Fig. 1d ). To exclude the possibility that co-localization of LINE-1 RNA with autophagosomes is an artifact of overexpression of LINE-1 fused with MS2-binding sites, we detected endogenous LINE-1 RNA using specific fluorescence in situ hybridization (FISH) probes recognizing retrotransposition-active LINE-1 elements of the L1-HS family ( Supplementary Fig. 1d,e ). Cytoplasmic foci of endogenous LINE-1 RNA also co-localized with LC3 ( Fig. 1e,f ). Three-dimensional-rendered Z-stacks of endogenous LINE-1 RNA and LC3 demonstrated that LINE-1 RNA is tightly associated with or enclosed within autophagosomes ( Fig. 1g ). 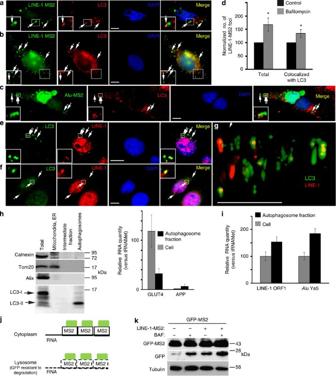Figure 1: LINE-1 andAluRNA are enclosed within autophagosomes. (a,b) Two representative images of fluorescent microscopy of LC3 and LINE-1 fused to six MS2-binding sites detected with MS2-GFP. (c) Fluorescent microscopy of LC3 andAlufused to six MS2-binding sites detected with MS2-GFP. Li’s correlation coefficient of co-localization (0.0232, s.e.m. 0.048). (d) Relative number of foci of LINE-1-MS2, or number of foci of LINE-1-MS2 co-localized with LC3 per cell in randomly selected fields of cells treated with BAF1 (20 h, 400 nM).n=25 cells, total number of LINE-1-MS2 foci: control=104, BAF=175, total number of LINE-1-MS2 foci co-localized with LC3: control =68, BAF 167. *TotalP=0.015, Co-localized with LC3P=5 × 10−8,t-test). Li’s correlation coefficient of co-localization (without BAF 0.19 s.e.m. 0.027; with BAF 0.213, s.e.m. 0.02). (e,f) Two representative images of fluorescent microscopy of FISH probes recognizing endogenous LINE-1 RNA and LC3. (g) Three-dimensional reconstruction of confocal microscopy z-stacks of endogenous LINE-1 RNA and LC3 prepared in Imaris. (h) Western blot of fractions enriched in autophagosomes compared with total cell extracts and ER/mitochondria-enriched fractions. RT-qPCR analysis of mRNA levels of two transmembrane proteins (GLUT4 and APP) in total cell RNA and autophagosome-enriched fractions.n=3,P>0.05. (i) RT-qPCR analysis of LINE-1 ORF1 andAluYa5in RNAse-treated autophagosome-enriched fractions or total cell RNA.n=3, *P=0.043 LINE-1,P-0.01AluYa5,t-test (j) Model of system to measure degradation of GFP-tagged substrates by autophagy. (k) Western blot analysis of GFP and alpha-tubulin (control) in cells transfected with MS2-GFP or LINE-1-MS2 and MS2-GFP and treated with control or Bafilomycin (2 h, 400 nM). All error bars represent s.e. of the mean. All experiments were replicated a minimum of three times. Figure 1: LINE-1 and Alu RNA are enclosed within autophagosomes. ( a , b ) Two representative images of fluorescent microscopy of LC3 and LINE-1 fused to six MS2-binding sites detected with MS2-GFP. ( c ) Fluorescent microscopy of LC3 and Alu fused to six MS2-binding sites detected with MS2-GFP. Li’s correlation coefficient of co-localization (0.0232, s.e.m. 0.048). ( d ) Relative number of foci of LINE-1-MS2, or number of foci of LINE-1-MS2 co-localized with LC3 per cell in randomly selected fields of cells treated with BAF1 (20 h, 400 nM). n =25 cells, total number of LINE-1-MS2 foci: control=104, BAF=175, total number of LINE-1-MS2 foci co-localized with LC3: control =68, BAF 167. *Total P =0.015, Co-localized with LC3 P =5 × 10 −8 , t -test). Li’s correlation coefficient of co-localization (without BAF 0.19 s.e.m. 0.027; with BAF 0.213, s.e.m. 0.02). ( e , f ) Two representative images of fluorescent microscopy of FISH probes recognizing endogenous LINE-1 RNA and LC3. ( g ) Three-dimensional reconstruction of confocal microscopy z-stacks of endogenous LINE-1 RNA and LC3 prepared in Imaris. ( h ) Western blot of fractions enriched in autophagosomes compared with total cell extracts and ER/mitochondria-enriched fractions. RT-qPCR analysis of mRNA levels of two transmembrane proteins (GLUT4 and APP) in total cell RNA and autophagosome-enriched fractions. n =3, P >0.05. ( i ) RT-qPCR analysis of LINE-1 ORF1 and AluYa5 in RNAse-treated autophagosome-enriched fractions or total cell RNA. n =3, * P =0.043 LINE-1, P -0.01 Alu Ya5, t -test ( j ) Model of system to measure degradation of GFP-tagged substrates by autophagy. ( k ) Western blot analysis of GFP and alpha-tubulin (control) in cells transfected with MS2-GFP or LINE-1-MS2 and MS2-GFP and treated with control or Bafilomycin (2 h, 400 nM). All error bars represent s.e. of the mean. All experiments were replicated a minimum of three times. Full size image Retrotransposon RNA co-purifies with autophagosomes As a first step to test whether LINE-1 and Alu RNA are enclosed within autophagosomes, these were purified [14] . The lipid-modified form of LC3 (LC3-II) that is specifically incorporated in autophagosomes was selectively enriched in these fractions compared with unmodified LC3-I ( Fig. 1h ). Autophagosome-enriched fractions were devoid of markers of other RNA-associated organelles such as mitochondria (TOM20), endoplasmic reticulum (Calnexin), endosomes and multivesicular bodies (Alix; Fig. 1h ). Autophagosome-enriched fractions were also not consistently enriched in mRNA of transmembrane proteins (APP, GLUT4), further excluding contamination with significant amounts of endoplasmic reticulum ( Fig. 1h ). Fractions enriched in intact autophagosomes were treated with RNAses to eliminate RNA attached to their external surface ( Supplementary Fig. 1f ). We measured the abundance of retrotransposon RNA by quantitative PCR with reverse transcriptase (RT-qPCR) using primers specific for active LINE-1 and Alu family members ( Supplementary Fig. 2 ). Autophagosome-enriched fractions contained abundant RNAse-protected LINE-1 (L1-HS) and Alu ( AluYa5 ) RNA compared with total cellular RNA by RT-qPCR ( Fig. 1i ). Together, this suggests that a substantial quantity of LINE-1 and Alu RNA is enclosed within autophagosomes. Retrotransposon RNA is degraded by autophagy Autophagosome content is degraded on fusion with lysosomes containing catabolic enzymes. GFP has an unusual resistance to proteolytic degradation in lysosomes; when GFP-tagged proteins are degraded by autophagy, a GFP fragment persists while the tagged protein is degraded ( Fig. 1j ) [15] . Background levels of free GFP were apparent in cells transfected with MS2-GFP alone ( Fig. 1k ). The expression of LINE-1 with MS2-binding sites markedly increased the amount of free GFP, and inhibiting lysosomal degradation with BAF caused GFP to accumulate further ( Fig. 1k ). This suggests that LINE-1 RNA with MS2-binding sites increases the recruitment of MS2-GFP into autophagosomes. Cumulatively, these data strongly suggest that LINE-1 RNA is enclosed within, and degraded by autophagosomes. If LINE-1 and Alu RNA are degraded by autophagy, they should accumulate when autophagy is inhibited. Either of the two independent siRNA-targeting ATG5 ( Supplementary Fig. 1a ), which is critical for autophagosome biogenesis, caused levels of LINE-1 (measured either at 5′UTR or ORF1), AluYa5 and AluYb8 RNA to increase ( Fig. 2a,b ). Alu inserts within longer RNAs are frequent [16] . We performed two tests to determine whether independent Alu elements were affected by autophagy. First, RNA was separated on gels and 250–350 nt RNAs consistent with the size of Alu were extracted and RT-qPCR was performed. Levels of AluYa5 and AluYb8 increased among 250–350 nt RNA in cells treated with ATG5 siRNA compared with control siRNA ( Fig. 2c , Supplementary Fig. 3a ). Second, RNA of ~300 nt detected by northern blot with probes for AluYa5 and AluYb8 also increased in cells treated with ATG5 siRNA compared with control siRNA ( Supplementary Fig. 3b ). This suggests that full-length Alu RNA accumulates when autophagy is inhibited, independent of longer RNAs containing Alu elements. LINE-1 and Alu RNA also accumulated when autophagic degradation was inhibited with BAF ( Supplementary Fig. 3c ). To ensure that increases in LINE-1 and Alu RNA levels when autophagy was inhibited were due to inhibited degradation and not activated transcription, we measured RNA decay using two assays. Blocking transcription with actinomycin D caused decay of LINE-1 and Alu Yb8 RNA that was impeded when autophagic degradation was blocked with Bafilomycin ( Fig. 2d , Supplementary Fig. 3d ). Decay of pulse-labelled LINE-1 and Alu Yb8 RNA was also inhibited in cells treated with ATG5 siRNA ( Fig. 2e , Supplementary Fig. 3e ). The majority of LINE-1 elements in the genome are drastically truncated at the 5′ end and inactive [5] , but RNA from 5′UTR and ORF1 of LINE-1 both accumulate when autophagy is inhibited ( Fig. 2a ). Cumulatively, this suggests that degradation of RNA from full-length, retrotransposition-competent LINE-1 and Alu is mediated by autophagy, in accord with its co-localization with and co-purification within autophagosomes ( Fig. 1 ). 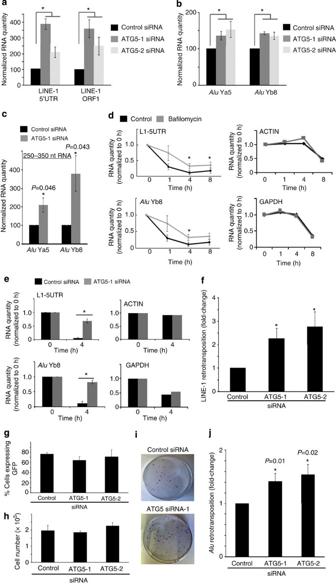Figure 2: Inhibiting autophagy increases levels of LINE-1 andAluRNA and their corresponding genomic insertions. (a,b) RT-qPCR analysis of levels of (a) LINE-1 RNA (5′UTR, ORF1,n=3, *P=0.009 LINE-1 5′UTR,P=0.03 LINE-1 ORF1,t-test) and (b)AluYa5andAluYb8in cells (n=3, *P=0.0018AluYa5,P=2 × 10−6AluYb8, analysis of variance (ANOVA)) treated with siRNA-targeting ATG5 or control (10 nM, 48 h) (c) RT-qPCR analysis ofAluYa5andAluYb8in 250–350 nt RNA isolated from cells treated with siRNA-targeting ATG5 or control (10 nM, 48 h,n=3, *P=0.046 AluYa5,P=0.043AluYb8, ANOVA). (d) RT-qPCR analysis in cells treated with dimethylsulphoxide or Bafilomycin (400 nM) and actinomycin D. (5 nM,n=3, *P=0.01 LINE-1 both 4 and 8 h,P=0.04AluYb8, ANOVA). (e) RT-qPCR analysis of pulse-labelled RNA recovered 0 and 4 h after pulse in cells transfected with siRNA-targeting ATG5 or control (10 nM,n=3, *P=0.01 both LINE-1 andAluYb8). (f) Percent of cells expressing GFP when co-transfected with LINE-1-RP GFP reporter of retrotransposition and siRNA-targeting ATG5 or control. Results are normalized to similar experiments with a retrotransposition-incompetent control (n=3, *P=0.045 ATG5-1,P=0.048 ATG5-2, ANOVA). (g) Relative number of cells at experiment’s termination if cells were transfected with siRNA-targeting ATG5 or control. (h) Percent of cells expressing GFP when co-transfected with plasmid expressing GFP and siRNA-targeting ATG5 or control (n=3). (i) Representative plates fromAlu-retrotransposition assay transfected with control siRNA or siRNA-targeting ATG5. (j) Relative number of G418-resistant colonies in cells transfected with siRNA-targeting ATG5 or control,Alu-retrotransposition reporter and retrotransposition-enhancer LINE-1 ORF2p (n=3, *P=0.01 ATG5-1,P=0.02 ATG5-2, ANOVA) All error bars represent s.e. of the mean. All experiments were performed with a minimum of three biological replicates. Figure 2: Inhibiting autophagy increases levels of LINE-1 and Alu RNA and their corresponding genomic insertions. ( a , b ) RT-qPCR analysis of levels of ( a ) LINE-1 RNA (5′UTR, ORF1, n =3, * P =0.009 LINE-1 5′UTR, P =0.03 LINE-1 ORF1, t -test) and ( b ) AluYa5 and AluYb8 in cells ( n =3, * P =0.0018 Alu Ya5, P =2 × 10 −6 Alu Yb8, analysis of variance (ANOVA)) treated with siRNA-targeting ATG5 or control (10 nM, 48 h) ( c ) RT-qPCR analysis of AluYa5 and AluYb8 in 250–350 nt RNA isolated from cells treated with siRNA-targeting ATG5 or control (10 nM, 48 h, n =3, * P =0.046 AluYa5, P =0.043 Alu Yb8, ANOVA). ( d ) RT-qPCR analysis in cells treated with dimethylsulphoxide or Bafilomycin (400 nM) and actinomycin D. (5 nM, n =3, * P =0.01 LINE-1 both 4 and 8 h, P =0.04 Alu Yb8, ANOVA). ( e ) RT-qPCR analysis of pulse-labelled RNA recovered 0 and 4 h after pulse in cells transfected with siRNA-targeting ATG5 or control (10 nM, n =3, * P =0.01 both LINE-1 and Alu Yb8). ( f ) Percent of cells expressing GFP when co-transfected with LINE-1-RP GFP reporter of retrotransposition and siRNA-targeting ATG5 or control. Results are normalized to similar experiments with a retrotransposition-incompetent control ( n =3, * P =0.045 ATG5-1, P =0.048 ATG5-2, ANOVA). ( g ) Relative number of cells at experiment’s termination if cells were transfected with siRNA-targeting ATG5 or control. ( h ) Percent of cells expressing GFP when co-transfected with plasmid expressing GFP and siRNA-targeting ATG5 or control ( n =3). ( i ) Representative plates from Alu -retrotransposition assay transfected with control siRNA or siRNA-targeting ATG5. ( j ) Relative number of G418-resistant colonies in cells transfected with siRNA-targeting ATG5 or control, Alu -retrotransposition reporter and retrotransposition-enhancer LINE-1 ORF2p ( n =3, * P =0.01 ATG5-1, P =0.02 ATG5-2, ANOVA) All error bars represent s.e. of the mean. All experiments were performed with a minimum of three biological replicates. Full size image Autophagy restricts retrotransposon insertion in the genome To test directly whether autophagic degradation targets active LINE-1 RNA and prevents new insertions of LINE-1 in the genome, we used an established LINE-1 retrotransposition reporter [13] . In this system, the LINE-1 that is expressed contains an intron with an inverted promoter and coding region for GFP [17] . When the LINE-1 is reverse transcribed and inserted into the genome, GFP is correctly oriented and can be expressed. Percent GFP+ cells are enumerated by flow cytometry [17] compared with cells transfected with GFP alone, or a GFP reporter with disabling mutations in LINE-1 (ref. 13 ). In these systems, effects on retrotransposition are usually measured by overexpressing a protein of interest. To evaluate more accurately the endogenous effect of autophagy on retrotransposition, we depleted cells of ATG5 using two independent siRNAs ( Supplementary Fig. 1a ). In cells depleted of ATG5, approximately twofold more cells expressed GFP, when transfected with active LINE-1 GFP-reporter compared with a control with point mutations that abolish retrotransposition ( Fig. 2f ) [12] . ATG5 knockdown did not affect cell number or transfection efficiency ( Fig. 2g,h ), suggesting that autophagic degradation of LINE-1 RNA quells retrotransposition of LINE-1 into the genome. To test the effect of autophagy on Alu retrotransposition, we utilized an established reporter designed similarly to the LINE-1 reporter, but substituting GFP expression for a geneticin resistance cassette [18] . In accord with abundant Alu RNA in autophagosome-enriched fractions ( Fig. 1i ), co-localization of Alu RNA to autophagosomes ( Fig. 1c ) and increased levels of Alu RNA on inhibition of autophagy ( Fig. 2b–e , Supplementary Fig. 3c ), depletion of ATG5 increased the number of resistant colonies obtained when cells were transfected with the Alu retrotransposition reporter compared with vector alone ( Fig. 2i,j ). Taken together, these results strongly suggest that degradation of LINE-1 or Alu RNA by autophagy restricts their genomic insertion. LINE-1 OR1p is also degraded by autophagy LINE-1 encodes ORF1p, an RNA-binding protein, which binds LINE-1 RNA in the cytoplasm and is required for LINE-1 retrotransposition [12] . GFP-ORF1p co-localized with the autophagosome marker LC3, and this co-localization increased when autophagy was inhibited ( Fig. 3a,b ). Endogenous ORF1p detected with a specific antibody ( Supplementary Fig. 4a ) also co-localized with LC3 ( Fig. 3c ) and was abundant in autophagosome-enriched fractions ( Fig. 3d ). Consistent with the autophagic degradation of ORF1p, free GFP accumulated in cells transfected with GFP-ORF1p when the cells were treated with BAF ( Fig. 3e ) [15] . This suggests that LINE-1 RNA is degraded by autophagy in complex with ORF1p. 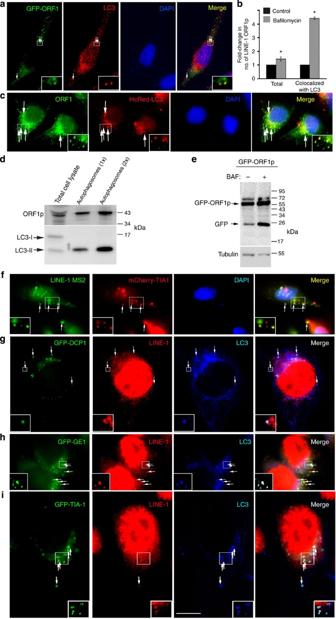Figure 3: LINE-1 RNA in P-bodies and stress granules co-localizes with autophagosomes and is likely degraded by autophagy with ORF1p. (a) Fluorescent microscopy of GFP-ORF1p and LC3. (b) Relative number of foci of GFP-ORF1p, or number of foci of GFP-ORF1p co-localized with LC3 per cell in randomly selected fields of cells treated with Bafilomycin A1 (20 h, 400 nM,n=30 cells, total number of GFP-ORF1p foci: control=150, BAF=214, total number of GFP-ORF1p co-localized with LC3: control=32, BAF=199). *P=0.007 Total,P=1 × 10−42Co-localized with LC3,t-test. Li’s correlation coefficient of co-localization (0.328, s.e.m. 0.019). Error bars represent s.e. of the mean. (c) Fluorescent microscopy of endogenous ORF1p and HcRed-LC3. (d) Western blot analysis of ORF1p in autophagosome-enriched fractions. LC3-II is a marker of autophagosomes. (e) Western blot analysis of GFP and alpha-tubulin (control) in cells transfected with GFP-ORF1p and treated with control or Bafilomycin (20 h, 400 nM). (f) Fluorescent microscopy of cells expressing LINE-1-MS2, MS2-GFP and mCherry-TIA-1. (g–i) Fluorescent microscopy of endogenous LINE-1 RNA in cells transfected with GFP-DCP1A (g), GFP-GE-1 (h) or GFP-TIA-1 (i). All experiments were performed with a minimum of three biological replicates. Figure 3: LINE-1 RNA in P-bodies and stress granules co-localizes with autophagosomes and is likely degraded by autophagy with ORF1p. ( a ) Fluorescent microscopy of GFP-ORF1p and LC3. ( b ) Relative number of foci of GFP-ORF1p, or number of foci of GFP-ORF1p co-localized with LC3 per cell in randomly selected fields of cells treated with Bafilomycin A1 (20 h, 400 nM, n =30 cells, total number of GFP-ORF1p foci: control=150, BAF=214, total number of GFP-ORF1p co-localized with LC3: control=32, BAF=199). * P =0.007 Total, P =1 × 10 −42 Co-localized with LC3, t -test. Li’s correlation coefficient of co-localization (0.328, s.e.m. 0.019). Error bars represent s.e. of the mean. ( c ) Fluorescent microscopy of endogenous ORF1p and HcRed-LC3. ( d ) Western blot analysis of ORF1p in autophagosome-enriched fractions. LC3-II is a marker of autophagosomes. ( e ) Western blot analysis of GFP and alpha-tubulin (control) in cells transfected with GFP-ORF1p and treated with control or Bafilomycin (20 h, 400 nM). ( f ) Fluorescent microscopy of cells expressing LINE-1-MS2, MS2-GFP and mCherry-TIA-1. ( g – i ) Fluorescent microscopy of endogenous LINE-1 RNA in cells transfected with GFP-DCP1A ( g ), GFP-GE-1 ( h ) or GFP-TIA-1 ( i ). All experiments were performed with a minimum of three biological replicates. Full size image LINE-1 RNA co-localizes with P-bodies and stress granules We next sought to determine how LINE-1 RNA is recruited to and degraded in autophagosomes. In accord with previous literature [11] , overexpressed LINE-1-MS2 RNA accumulated in stress granules ( Fig. 3f ). In contrast, endogenous LINE-1 RNA co-localized strongly with markers of P-bodies, which concentrate RNA decay enzymes (GFP-DCP1A or GFP-Ge-1, Fig. 3g,h ), and to a lesser extent with stress granules (GFP-TIA-1, Fig. 3i ). A similar localization of endogenous LINE-1 RNA was observed when P-bodies and arsenite-induced stress granules were detected with antibodies to endogenous proteins (Rck, TIAR, Supplementary Fig. 4b,c ). LINE-1-MS2 also co-localized in part with arsenite-induced stress granules ( Supplementary Fig. 4d ). LINE-1 RNA that co-localized with GFP-DCP1A or GFP-TIA-1 also co-localized with LC3 ( Fig. 3g–i ), suggesting that LINE-1 RNA in either stress granules or P-bodies can be targeted for autophagic degradation. Autophagy receptors help selectively degrade RNA granules Selective autophagy receptors, such as NDP52 and p62, recruit nascent autophagosome membranes to substrates of autophagy [2] . NDP52 or p62, labelled with specific antibodies ( Supplementary Fig. 5a,b ), co-localized with foci of endogenous LINE-1 RNA, LINE-1-MS2 ( Fig. 4a–d ) and Alu- MS2 ( Supplementary Fig. 5c,d ). In four-colour confocal microscopy, exclusive markers of stress granules (mCherry-TIA-1) and P-bodies (GFP-DCP1A) were often adjacent, but not co-localized as expected [19] ( Fig. 4e ). p62 preferentially co-localized with mCherry-TIA-1 compared with NDP52, while NDP52 preferentially co-localized with GFP-DCP1A ( Fig. 4e,f ). NDP52 co-localized with a small proportion of stress granules ( Fig. 4f,g ), but p62 was always also present in these stress granules ( Fig. 4h ). Similarly, p62 co-localized with a small proportion of P-bodies, but NDP52 was virtually always co-present ( Fig. 4e–h ). A third autophagy receptor, NBR1, also co-localized with a subset of P-bodies ( Supplementary Fig. 5e,f ). NDP52 and p62 also preferentially co-localized with markers of endogenous P-bodies (GW182) and arsenite-induced stress granules (DDX3), respectively ( Supplementary Fig. 6a–e ). This suggests that p62 and NDP52 are preferentially recruited to stress granules and P-bodies, respectively, which frequently co-localize with autophagosomes ( Fig. 3g–i ). 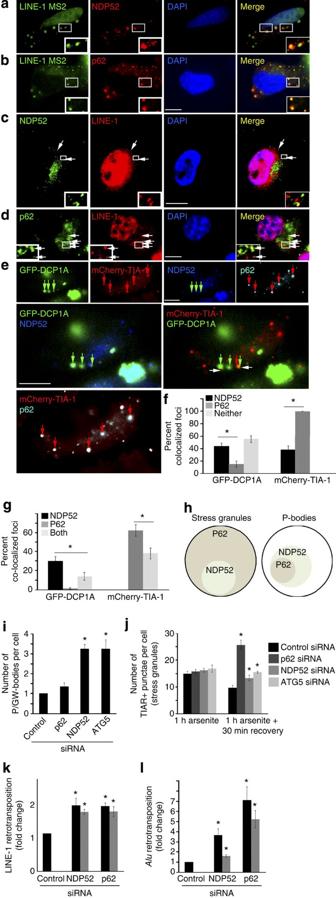Figure 4: LINE-1 RNA in P-bodies or stress granules is preferentially targeted for autophagic degradation by NDP52 and P62, respectively. (a,b) Fluorescent microscopy of (a) NDP52 or (b) P62 in cells expressing LINE-1-MS2 and MS2-GFP. (c,d) Fluorescent microscopy of endogenous LINE-1 RNA and (c) NDP52 or (d) P62. (e) Four-colour confocal microscopy of NDP52, P62, GFP-DCP1A and mCherry-TIA-1. (f) Percent of foci of NDP52, P62 or neither co-localizing with GFP-DCP1A or mCherry-TIA-1. *P=0.007 GFP-DCP1A,P=0.00005 mCherry-TIA-1, analysis of variance (ANOVA). (g) Percent of foci of NDP52, P62 or both co-localizing with GFP-DCP1A or mCherry-TIA-1,n=674 stress granules,n=53 P-bodies. *P=0.043 GFP-DCP1A,P=0.028 mCherry-TIA-1, ANOVA. (h) Venn diagram of the percent of P-bodies (GFP-DCP1A) or stress granules (mCherry-TIA-1) co-localizing with NDP52, P62, both or neither. (i) Relative number of P-bodies per cell (detected with 18033 serum-recognizing GW182) treated with indicated siRNAs.n=3, *P=0.0002 NDP52,P=0.004 ATG5. (j) Relative number of stress granules (detected with antibody recognizing TIAR) 1 h after arsenite treatment and after 30 min recovery from 1 h treatment with arsenite.n=3, *P=4x10−6p62,P=0.019 NDP52,P=2 × 10−5ATG5, ANOVA. (k) Percent of cells expressing GFP when co-transfected with LINE-1-RP retrotransposition GFP reporter and either of two independent siRNA (black and grey bars) targeting NDP52, P62 or control. Results are normalized to a retrotransposition-incompetent control (n=3, *P=0.017,P=0.002 NDP52;P=0.001,P=0.013 p62, ANOVA). (l) Relative number of G418-resistant colonies in cells transfected with siRNA-targeting NDP52, P62 or control,Alu-retrotransposition reporter and retrotransposition-enhancer LINE-1 ORF2p (n=3, *P=0.012,P=0.011 NDP52;P=0.008,P=0.011 p62, ANOVA). All error bars represent s.e. of the mean. All experiments were performed with a minimum of three biological replicates. Figure 4: LINE-1 RNA in P-bodies or stress granules is preferentially targeted for autophagic degradation by NDP52 and P62, respectively. ( a , b ) Fluorescent microscopy of ( a ) NDP52 or ( b ) P62 in cells expressing LINE-1-MS2 and MS2-GFP. ( c , d ) Fluorescent microscopy of endogenous LINE-1 RNA and ( c ) NDP52 or ( d ) P62. ( e ) Four-colour confocal microscopy of NDP52, P62, GFP-DCP1A and mCherry-TIA-1. ( f ) Percent of foci of NDP52, P62 or neither co-localizing with GFP-DCP1A or mCherry-TIA-1. * P =0.007 GFP-DCP1A, P =0.00005 mCherry-TIA-1, analysis of variance (ANOVA). ( g ) Percent of foci of NDP52, P62 or both co-localizing with GFP-DCP1A or mCherry-TIA-1, n =674 stress granules, n =53 P-bodies. * P =0.043 GFP-DCP1A, P =0.028 mCherry-TIA-1, ANOVA. ( h ) Venn diagram of the percent of P-bodies (GFP-DCP1A) or stress granules (mCherry-TIA-1) co-localizing with NDP52, P62, both or neither. ( i ) Relative number of P-bodies per cell (detected with 18033 serum-recognizing GW182) treated with indicated siRNAs. n =3, * P =0.0002 NDP52, P =0.004 ATG5. ( j ) Relative number of stress granules (detected with antibody recognizing TIAR) 1 h after arsenite treatment and after 30 min recovery from 1 h treatment with arsenite. n =3, * P =4x10 −6 p62, P =0.019 NDP52, P =2 × 10 −5 ATG5, ANOVA. ( k ) Percent of cells expressing GFP when co-transfected with LINE-1-RP retrotransposition GFP reporter and either of two independent siRNA (black and grey bars) targeting NDP52, P62 or control. Results are normalized to a retrotransposition-incompetent control ( n =3, * P =0.017, P =0.002 NDP52; P =0.001, P =0.013 p62, ANOVA). ( l ) Relative number of G418-resistant colonies in cells transfected with siRNA-targeting NDP52, P62 or control, Alu -retrotransposition reporter and retrotransposition-enhancer LINE-1 ORF2p ( n =3, * P =0.012, P =0.011 NDP52; P =0.008, P =0.011 p62, ANOVA). All error bars represent s.e. of the mean. All experiments were performed with a minimum of three biological replicates. Full size image Previous work demonstrated that stress granules and P-bodies can be degraded by autophagy [3] . NDP52 selectively localized with P-bodies ( Fig. 4e–h , Supplementary Fig. 6a–d ) and the knockdown of NDP52, but not p62, caused a marked increase in the number of P-bodies per cell ( Fig. 4i , Supplementary Fig. 7a ). Similarly, p62 selectively labelled stress granules ( Fig. 4e–h , Supplementary Fig. 6a–d ) and knockdown of p62, and to a lesser extent NDP52, caused a marked increase in stress granules in cells during recovery from arsenite-induced stress ( Fig. 4j , Supplementary Fig. 7b,c ). This suggests that p62 and NDP52 selectively target stress granules and P-bodies, respectively, for degradation by autophagy. NDP52 and p62 exhibited more co-operative effects on number of P-bodies labelled with GFP-Dcp1a and stress granules induced by the overexpression of mCherry-TIA-1 ( Supplementary Fig. 7d,e ). This closely resembles targeting of bacteria invading the cytoplasm in which p62 and NDP52 are also recruited independently, but collaboratively target bacteria for autophagic engulfment [20] . NDP52 and p62 limit genomic insertions of retrotransposons Knockdown of p62 or NDP52 ( Supplementary Fig. 5a,b ) increased the levels of LINE-1 and Alu RNA ( Supplementary Fig. 8a,b ). Independent Alu elements of 250–350 nt also increased in cells depleted of NDP52 or p62 with siRNA ( Supplementary Figs 3a and 8c,d ). Knockdown of p62 or NDP52 also increased the rates of genomic insertion of LINE-1 and Alu ( Fig. 4k,l , Supplementary Fig. 8e,f ). Together, this suggests that p62 and NDP52 selectively target stress granules and P-bodies containing retrotransposon RNA for degradation by autophagy, thereby preventing the insertion of LINE-1 and Alu into the genome. Beclin1/Atg6 mice accumulate retrotransposon insertions BECLIN1/ATG6 ( BECN1/ATG6) , a gene required for autophagosome biogenesis [21] , is lost in 40–70% of human breast and ovarian cancer patients [22] . To examine whether Becn1/Atg6 controls LINE-1 activity in a controlled system, we used Becn1/Atg6 +/− mice. Levels of LINE-1 RNA increased in ovaries of Becn1/Atg6 +/− mice compared with wild type ( Fig. 5a ). We tested the relative number of LINE-1 genomic insertions using an established qPCR assay that is specific for the small number of active LINE-1 (approximately 1,290) and faithfully mirrors rates of insertion analysed by genome sequencing [6] , [7] . Importantly, this assay measures the relative quantity of ORF2 (3′ of LINE-1) normalized to the 5′UTR of LINE-1, which is truncated in virtually all new LINE-1 insertions [5] . This ensures that de novo insertions of LINE-1 are measured rather than unrelated chromosomal amplification. In Becn1/Atg6 +/− mice, the relative number of LINE-1 insertions increased in the ovary (13%, Fig. 5b ) compared with the wild-type controls. This represents approximately 150 new insertions per cell in the ovary, in the range of LINE-1 insertions observed during neurogenesis [23] . Other studies had observed higher rates of LINE-1 insertions in brain and muscle than in liver and other tissues [23] , [24] . Screening other tissues for LINE-1 activity in Becn1/Atg6 +/− mice, we observed that the levels of LINE-1 RNA increased in the prefrontal cortex ( Fig. 5c ). Levels of genomic insertions of LINE-1 increased in prefrontal cortex and muscle, but not liver ( Fig. 5c,d ). This suggests that Atg6/Becn1 and autophagy control retrotransposon RNA levels and retrotransposon-mediated genetic change in mice. 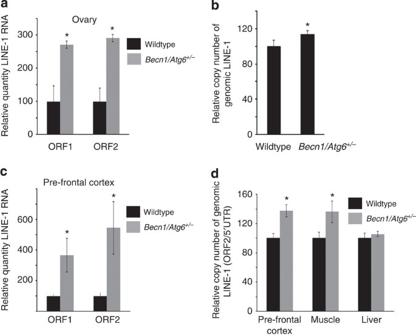Figure 5: Levels of LINE-1 RNA and genomic insertions increase in mice with loss ofBecn1/Atg6. (a) RT-qPCR analysis of the levels of LINE-1 ORF1 and ORF2 RNA in ovaries ofBecn1/Atg6+/−mice compared with wild-type controls (n=4 wild-type,Becn1/Atg6+/−mice). (b) qPCR analysis of relative number of genomic copies of LINE-1 ORF2 in ovaries ofBecn1/Atg6+/−mice and wild-type controls normalized to LINE-1 5′UTR and 5S rDNA (n=4 wild-type, 6Becn1/Atg6+/−mice). *P=0.02,t-test. (c) RT-qPCR analysis of the levels of LINE-1 ORF1 and ORF2 RNA in the prefrontal cortex ofBecn1/Atg6+/−mice compared with wild-type controls (n=4 wild-type,Becn1/Atg6+/−mice). (d) qPCR analysis of relative number of genomic copies of LINE-1 ORF2 in muscle, liver and prefrontal cortex ofBecn1/Atg6+/−mice and wild-type controls normalized to LINE-1 5′UTR and 5S rDNA (n=4 wild-type, 6Becn1/Atg6+/−mice). *P=0.019 prefrontal cortex,P=0.048 muscle, analysis of variance. All error bars represent s.e. of the mean. Figure 5: Levels of LINE-1 RNA and genomic insertions increase in mice with loss of Becn1/Atg6 . ( a ) RT-qPCR analysis of the levels of LINE-1 ORF1 and ORF2 RNA in ovaries of Becn1/Atg6 +/− mice compared with wild-type controls ( n =4 wild-type, Becn1/Atg6 +/− mice). ( b ) qPCR analysis of relative number of genomic copies of LINE-1 ORF2 in ovaries of Becn1/Atg6 +/− mice and wild-type controls normalized to LINE-1 5′UTR and 5S rDNA ( n =4 wild-type, 6 Becn1/Atg6 +/− mice). * P =0.02, t -test. ( c ) RT-qPCR analysis of the levels of LINE-1 ORF1 and ORF2 RNA in the prefrontal cortex of Becn1/Atg6 +/− mice compared with wild-type controls ( n =4 wild-type, Becn1/Atg6 +/− mice). ( d ) qPCR analysis of relative number of genomic copies of LINE-1 ORF2 in muscle, liver and prefrontal cortex of Becn1/Atg6 +/− mice and wild-type controls normalized to LINE-1 5′UTR and 5S rDNA ( n =4 wild-type, 6 Becn1/Atg6 +/− mice). * P =0.019 prefrontal cortex, P =0.048 muscle, analysis of variance. All error bars represent s.e. of the mean. Full size image Autophagy is a selective, stress-enhanced mechanism for degrading specific cytoplasmic contents. Despite critical roles for autophagy in cancer and several other diseases, surprisingly little is known about RNA degradation by autophagy. Data presented here strongly suggest that retrotransposon RNA is degraded by autophagy, and that impeding this process causes accumulation of retrotransposon RNA and genomic insertions. Evidence to date suggests that RNAs are targeted for autophagic degradation as part of RNA granules such as stress granules [3] , [25] . Autophagy may be a more efficient mechanism for disposing of such large clusters of RNA than canonical RNA degradation complexes. Our evidence demonstrates that NDP52 preferentially localizes to P-bodies, while p62 preferentially localizes to stress granules, suggesting that autophagy can selectively target distinct RNA granules. Intriguingly, emerging evidence suggests that pathology in amyotrophic lateral sclerosis involves inhibited autophagic degradation of mutant proteins like TDP43 and FUS in stress granules [3] . Our identification of p62 as a selective autophagy receptor for degradation of stress granules suggests a mechanism for the genetic implication of p62 in amyotrophic lateral sclerosis [26] . Levels of LINE-1 RNA and genomic insertions also increase when a copy of the autophagy-critical gene Becn1/Atg6 is lacking in mice, suggesting that the loss of BECN1/ATG6 , which is common in ovarian, breast and prostate cancers may lead to LINE-1-induced genetic instability. A previous study demonstrated that BECN/ATG61 +/− cells exhibit genetic instability and marks of DNA damage responses for unknown reasons [27] . LINE-1 and Alu retrotransposons instigate much more chromosomal instability than their insertions alone; LINE-1 ORF2p endonuclease activity generates double-stranded DNA breaks in great excess of those required for reinsertion of LINE-1 into the genome [28] . LINE-1 and Alu are also a frequent cause of interchromosomal translocations, intrachromosomal deletions, inversions and amplifications [29] , [30] , [31] . This suggests that unmoderated LINE-1 activity could contribute to the genomic instability caused by the lack of autophagy in BECN1/ATG6 +/− cells [27] . Interestingly, only 15% of BECN1/ATG6 +/− mice develop tumours [21] suggesting that the underlying process is stochastic, like the insertion of retrotransposons into the genome. Mechanisms that promote genetic or epigenetic diversity in response to stress may be favoured by evolution [32] . Proteins that suppress retrotransposons can act as capacitors or buffers of phenotypic diversity [33] . Many stresses induce transcription of retrotransposons and may promote somatic or inherited genetic change [34] . Our results suggest that autophagy, as a stress-induced response, tempers somatic variegation and evolutionary change by degrading retrotransposon RNA. RT-qPCR RT-qPCR was performed with the MiScript II Reverse Transcriptase system (Qiagen) and GoTaq qPCR Master Mix (Promega A6002). The following primers were used, as described [23] to quantify RNA in human cells: L1-ORF1: 5′-TCA AAG GAA AGC CCA TCA GAC TA-3′, 5′-TGG CCC CCA CTC TCT TCT-3′; L1-5UTR: 5′-ACG GAA TCT CGC TGA TTG CTA-3′, 5′-AAG CAA GCC TGG GCA ATG-3′; Alu-Sg: 5′-TTC GAG ACC AGC CTG GCC-3′, 5′-CT CCC GGG TTC AAG CGA-3′; Alu-Ya5: 5′-TCC CGG CTA AAA CGG TGA AA-3′, 5′-CTC CCA AGT AGC TGG GAC TAC AGG-3′; Alu-Yb8: 5′-ATC CTG GCT AAC AAG GTG AAA CCC-3′, 5′-CGG ACT GCT GGA CTG CAG TG-3′, β-actin: 5′-GGCATGGGTCAGAAGGATT- 3′ and 5′-GGGGTGTTGAAGGTCTCAAA-3′; GAPDH: 5′-ATC TTC TTG TGC AGT GCC AG-3′, 5′-TTT GCC ACT GCA AAT GGC AG-3′ For RT-qPCR of mouse tissues, primers were designed as described [23] : 18S: 5′-ATG GTA GTC GCC GTG CCT AC-3′; 5′-CCG GAA TCG AAC CCT GAT T-3′; mL1-ORF1a: 5′-ACT CAA AGC GAG GCA ACA CTA GA-3′; 5′-GTT CCA GAT TTC TTT CCT AGG GTT TC-3′; mL1-ORF1b: 5′-AGG CTA CTA TAC CCA GCC AAA CTC T-3′; 5′-TAC TTT GGT TTC TCC CTC TAT GAT AAT TG-3′; mL1-ORF2a: 5′-CCT CCA TTG TTG GTG GGA TT-3′;5′-GGA ACC GCC AGA CTG ATT TC-3′; mL1-Orf2b: 5′-CTG GCG AGG ATG TGG AGA A-3′; 5′-CCT GCA ATC CCA CCA ACA AT-3′. Relative quantities were calculated using the ΔΔ C t method, normalizing to the geometric mean of β-actin and GAPDH. qPCR of genomic LINE-1 Quantification of genomic insertions of LINE-1 was performed as described [6] , [23] . Briefly, genomic DNA was isolated using GenElute Mammalian Genomic DNA Miniprep kits (Sigma, G1N70-1KT), which includes RNAse A treatment of genomic DNA. LINE-1 ORF2, 5′UTR or 5S rRNA were amplified in quadruplicate with the polymerase and primers previously described [23] using GoTaq qPCR Master Mix (Promega A6002). We calculated the percent increase in LINE-1 insertions as described [6] , [23] . LINE-1 insertions are overwhelmingly (~99%) and severely truncated at the 5′ end; therefore, the relative number of new insertions are estimated in this method normalizing LINE-1 ORF2 (3′) to LINE-1 5′UTR and 5S (ref. 23 ) to avoid measuring genomic amplification due to other effects than LINE-1 insertion. Cells and reagents HeLa (CCL2, ATCC), 293T cells (CRL-3216, ATCC) were cultured in Dulbecco’s Modified Eagle’s Medium containing 10% fetal bovine serum and 2 mM L -glutamine. The following plasmids were gifts from J. Goodier (John Hopkins): GFP-MS2 (ref. 35 ), LINE-1-MS2 (ref. 36 ), Alu-MS2 (ref. 36 ) and GFP-ORF1p (ref. 37 ). GFP-Dcp1a (gift from W. Filipowicz, Freidrich Miescher Institute), GFP-Ge-1 (ref. 38 ) and TIA-mCherry (gift from J. Cote, University of Ottawa) were also used. The following primary antibodies were used in this study: LC3 (Cell Signaling #2775), ORF1p (ref. 39 ) (a kind gift from C. Harris, University of Medicine and Dentistry of New Jersey), DICER (clone 13D6, Santa Cruz), NDP52 (ab688588), P62 (clone 3, BD Biosciences), DDX3 (A300-474A, Bethyl Labs), FMRP (clone 1C3, Millipore), TIAR (Cell Signaling Technology), Rck (#9407, Cell Signaling Technology), TOM20 (clone FL-145, Santa Cruz), Calnexin (polyclonal, Stressgen) and Alix (clone 2H12, Santa Cruz) and serum 18033 recognizing GW182 (ref. 40 ) (a kind gift from M. Fritzler, University of Calgary). All antibodies were used at 1/500 dilutions. Silencer Select siRNAs (Life Technologies) were transfected with RNAiMax (Life Technologies). The siRNAs used were: ATG5 5′-AUAUCUCAUCCUGAUAUAGCgt-3′ (siRNA ID s18160) and 5′-AUGAGCUUCAAUUGCAUCCtt-3′ (siRNA ID s18158), P62 5′-siRNAUUUAAUGUAGAUUCGGAAGat-3′ (siRNA ID s16962) and 5′-UCUUUUCCCUCCGUGCUCCac-3′ (siRNA ID s16960) and NDP52 5′-siRNAAAAGUAACCCACAUGAAGGtg-3′ (siRNA ID s19996) and 5′-UUUGUUGUUUAGGUCAAUGgg-3′ (siRNA ID s19994). Gel extraction of RNA for RT-qPCR of Alu RNA RNA was separated on a 6% acrylamide gel and stained with ethidium bromide. The region between 250 and 350 nucleotides was excised with a scalpel and incubated with 400 μl of gel elution buffer (20 mM Tris–HCl, 0.25 M sodium acetate, 1 mM EDTA, 0.25% SDS, pH 7.5). The mixture was frozen on dry ice for 15 min and incubated at room temperature overnight to allow RNA to diffuse from the gel. The mixture was subsequently centrifuged at 21,000 g for 10 min at room temperature. The supernatant was retrieved for RNA purification with Trizol reagent (Invitrogen). Pulse labelling of RNA with ethynyl uridine Pulse labelling was performed with Click-iT technology using the Nascent RNA Click-iT kit (Life Technologies) according to manufacturer’s instructions. Briefly, cells were plated at 2.5 × 10 5 per well in a six-well plate and transfected with siRNA the following day. Forty-eight hours after tranfection, ethynyl uridine (0.2 mM) was added. Media was changed after 1 h incubation and RNA was extracted immediately or after four more hours using Trizol reagent. Ethynyl uridine incorporated in RNA (5 μg) was labelled with biotin (0.5 mM biotin azide per sample). Pulse-labelled, biotinylated RNA (500 ng) was captured using Dynabeads Streptavidin T1 magnetic beads and used as a template for cDNA synthesis using SuperScript VILO cDNA Synthesis Kit (Life Technologies). RNA decay with actinomycin D Cells were plated in six-well plates at a concentration of 2.5 × 10 5 per well. Dimethylsulphoxide or Bafilomycin (400 nM, Millipore) were added to wells for 30 min, then Actinomycin D (Sigma-Aldrich) was added at a final concentration of 5 μg ml −1 . RNA was extracted from cells immediately or 1, 4 or 8 h later using TRI reagent (Sigma, T9424-200ML), cDNAs were synthesized using SuperScript VILO cDNA Synthesis Kit (Invitrogen, 11754-250). Alu retrotransposition assay Retrotransposition assay was performed as described [18] , [36] . In brief, 5 × 10 3 cells were plated in a 60-mm dish. The following day, Alu -neo Tet (refs 18 , 36 ) was co-tranfected with the retrotransposition driver plasmid pCEP 5′UTR ORF2-no neo [41] or pcDNA3.1 (control) and 10 nM of siRNA using Lipofectamine 2000 (Invitrogen). SiRNA alone was transfected as an additional control for selection. One week after transfection, the cells were counted and 5 × 10 3 cells were replated in 100 mm plates. The second day after replating, 600 μg ml −1 G418 (Life Technologies) was added and replaced every 3 days. After 10 days of selection, colonies were stained with crystal violet (Sigma-Aldrich), and counted. LINE-1 retrotransposition assay Retrotransposition assays were performed as described [36] . Briefly, 2.5 × 10 5 cells per well were seeded in six-well dishes. The next day, 1.0 μg of 99 RPS-GFP PUR, containing LINE-1-RP coupled with an enhanced GFP retrotransposition reporter cassette or 99 RPS-GFP JM111 PUR, containing LINE-1-RP with two point mutations in ORF1 that abolish retrotransposition [12] (gifts from J. Goodier) [36] , [42] , was co-transfected together with 10 nM of siRNA using Lipofectamine 2000 (Invitrogen). All transfections were in triplicate. Five days post transfection, percent GFP-expressing cells was measured by flow cytometry (FC500, Beckman Coulter). To account for the effects of siRNA-mediated knockdown on transfection efficiency, or cell proliferation/death, independent cells were transfected with enhanced GFP-N1-expressing plasmid. Fluorescence microscopy Cells were prepared for microscopy as previously described [4] , [43] . Cells were grown on 0.17-mm glass coverslips overnight before fixation in 2% paraformaldehyde in PBS (10 min). Cells were rinsed twice in PBS and incubated for 10 min with 0.2% Triton-X-100 in PBS and 20 mM NH 4 Cl. After washing with PBS, cells were blocked with 5% milk in PBS (1 h), washed three times in PBS and incubated with 5 μg ml −1 primary antibody overnight at 4 °C, washed three times (10 min) in PBS and incubated with 1/300 dilution of highly cross-adsorbed secondary antibodies (goat anti-mouse Alexa488 or -633, anti-rabbit Alexa 488 or -546 (Invitrogen) or anti-rabbit DyLight 405 (Jackson Immunoresearch)) for 1 h. After washing three times (10 min), cells were mounted with Vectashield Mounting Media and imaged on a Zeiss AxioObserver Z1 or a Zeiss 510 confocal microscope. Endogenous LINE-1 RNA was labelled using 48 Quasar570-labelled probes designed and produced by Biosearch Technologies (Petaluma, CA, USA). The sequence of L1 probes was: 5′-TTTGTTTACCTAAGCAAGCC-3′, 5′-CTGTCTTTTTGTTTGTCTGT-3′, 5′-CACTTAAGTCTGCAGAGGTT-3′, 5′-CTCTCTTCAAAGCTGTCAGA-3′, 5′-ATGGGTTTTCGGTGTAGATG-3′, 5′-TCTTTGCCTTTGGTTTGAAT-3′, 5′-AAGCACTTCTCTGTATTGGT-3′, 5′-CATTCTTCACGTAGTTCTCG-3′, 5′-ATATTTCTTGGAGGCTTTGC-3′, 5′-GGGAAGTTCTCCTGGATAAT-3′, 5′-TTGATGCAGTTTCTTCCTAG-3′, 5′-CCCATTATTAATGTGTGGGA-3′, 5′-TAATGTTGACAGTGGGGTGT-3′, 5′-TTGACTTTCTGTCTCGTTGA-3′, 5′-AGAGCTGAGTTCAATTCCTG-3′, 5′-AGATGTCTATTAGGTCTGCT-3′, 5′-TAGTTTGATTGCACTGTGGT-3′, 5′-TATGTGGTGTCTTTGTTCTC-3′, 5′-AATTTTGGATCTTTCCTGCT-3′, 5′-AATGTGTTTGCTCTTGCTTT-3′, 5′-TTTGTGTCTCTATTTCCTTC-3′, 5′-TGCTAGCGGTCTATCAATTT-3′, 5′-TTTGCGTAGAGGTGTTTGTA-3′, 5′-CTTTTTTGGTTGTGTCTCTG-3′, 5′-GTCAAAGGCTTTTTCTGCAT-3′, 5′-GTGGGTTTGTCATAGATAGC-3′, 5′-AAGGGAATGCTTCCAGTTTT-3′, 5′-AATACCCTTTATTTCCTTCT-3′, 5′-AGGGACAATTTGACTTCCTC-3′, 5′-TTCACATCCCTTGTAAGTTG-3′, 5′-TTTATTTCCTTGAGCAGTGG-3′, 5′-TTCTTCCATTTGTTTGTGTC-3′, 5′-CTTTGTTCTTTTGGCTTAGG-3′, 5′-GAAGTCAGGTAGTGTGATGC-3′, 5′-AAGGAAGGGATCCAGTTTCA-3′, 5′-CTGAATGGTAATGCCTAGGT-3′, 5′-ATGGTAGTTTCTTTTGCTGT-3′, 5′-GCGAAAATTTTCTCCCATGT-3′, 5′-CACTTTTTGATGGGGTTGTT-3′, 5′-ATGTGTTTTTTGGCTGCATA-3′, 5′-CCATTCTAACTGGTGTGAGA-3′, 5′-CCCACCAACAGTGTAAAAGT-3′, 5′-CACACTGACTTCCACAATGG-3′, 5′-GGTATATACCCAGTAATGGG-3′, 5′-CGTGTGCATGTGTCTTTATA-3′, 5′-CCAAGTCTTTGCTATTGTGA-3′, 5′-TCATTGTTGGACATTTGGGT-3′, 5′-TATGCGGTGTTTGGTTTTTT-3′. For labelling with FISH probes, cells were fixed in 1% formaldehyde in PBS for 10 min, washed twice in PBS, permeabilized with 0.2% Triton-X-100 (7 min), washed again and incubated (5 min) in 10% formamide in 2 × SSC buffer. Subsequently, 3 μM of LINE-1 FISH probes and 2.5 μg ml −1 of LC3 antibody were incubated with cells overnight at 37 °C in hybridization buffer (0.1% Triton-X-100, 0.1% Tween-20, 100 mg ml −1 dextran sulfate and 10% formamide in 2 × SSC). Sections were incubated with secondary antibody (1 h), washed with PBS and mounted. Quantification of microscopy Image fields were randomly selected. The number of stress granules (labelled with anti-TIAR antibody) and P-bodies (labelled with 18033 serum-recognizing GW182) were quantified using the automatic particle counting tool of ImageJ. To distinguish particles of interest from background with minimal user bias, a threshold range was calculated using Li’s Minimum Cross Entropy method [44] . Binary images were obtained on applying the threshold settings (see Supplementary Fig. 6c ). Pixel area size was set to 0.05–10 μm to exclude the nuclear staining of TIAR and foci were counted using the Analyze Particles function of ImageJ. The total number of stress granules or P-bodies was then divided by the number of cells. To calculate the number of P-bodies (GFP-Dcp1a) or stress granules (mCherry-TIA-1) per cell, the total number of each was counted per cell, based on DAPI (4,6-diamidino-2-phenylindole) staining and differential interference contrast images. In Fig. 4f , each P-body (GFP-Dcp1a) or stress granule (mCherry-TIA-1) in a cell was counted as being co-localized with p62, NDP52 or neither p62 or NDP52/total number of P-bodies or stress granules in the cell. In Fig. 4g , each P-body (GFP-Dcp1a) or stress granule (mCherry-TIA-1) in a cell was counted as being co-localized with p62 alone, NDP52 alone or both p62 and NDP52/total number of P-bodies or stress granules in the cell. P-bodies or stress granules co-localizing with neither are not included in Fig. 4g . Coefficients of co-localization were calculated using Just Another Co-localization Plugin [45] . Autophagosome purification Autophagosomes were fractionated essentially as described [14] . Twenty 160 cm 2 plates of 293 cells were harvested into 0.25 M sucrose 10 mM HEPES pH 7.2, washed several times in the same solution, transferred into 0.25 M sucrose containing protease inhibitor cocktail (Roche, EDTA-free) and disrupted by nitrogen cavitation (Parr Instruments, 100 p.s.i. 30 s, 50 p.s.i. 30 s, 25 p.s.i. 8 min). Lysate was centrifuged twice at 2,000 g to eliminate intact cells and large debris. Supernatant was then centrifuged at 17,000 g (12 min) to pellet organelles. The pellet was resuspended in 0.25 M sucrose 10 mM HEPES pH 7.2 and treated with a mixture of RNAse A/T1 (Fermentas) for 10 min, 37 °C. Organelles were then loaded at the bottom of a discontinuous Histodenz density gradient (26, 24, 20 and 15%) and centrifuged at 90,000 g for 3 h in an SW41 rotor (Beckman). Fractions at the interface of 15–20% and 20–24% densities are enriched in autophagosomes and autophagolysosomes, respectively. Autophagosome-enriched fractions were used for all analyses. Analysis of Becn1/Atg6 +/− mice All experiments were approved by the University of Ottawa Animal Care Committee according to Canadian Council on Animal Care guidelines. Four-week-old Becn1/Atg6 +/− female mice and wild-type littermates from two independent litters were killed and ovaries, prefrontal cortex, muscle and liver were harvested, flash frozen in liquid nitrogen and stored at −80 °C before analysis as above. Analysis was not blinded. Statistics Two-tailed t -tests or analysis of variance were employed to evaluate the statistical significance of RT-qPCR, retrotransposition and microscopy quantifications on a minimum of three independent biological replicates. How to cite this article : Guo, H. et al. Autophagy supports genomic stability by degrading retrotransposon RNA. Nat. Commun. 5:5276 doi: 10.1038/ncomms6276 (2014).